Visualization of caspase-3-like activity in cells using a genetically encoded fluorescent biosensor activated by protein cleavage Cytosolic caspase-3-like proteases, such as caspase-3 and caspase-7, have a central role in mediating the progress of apoptosis. Here to conveniently monitor caspase-3-like activity in the multicellular environment, we have developed genetically encoded switch-on fluorescence-base indicators that are cyclized chimeras containing a caspase-3 cleavage site as a switch. When cleaved by caspase-3-like proteases, the non-fluorescent indicator rapidly becomes fluorescent, and thus detects in real-time the activation of such caspases. We generate cultured cells constitutively expressing these chimeras, and all the healthy cells are non-fluorescent. When these cells are exposed to apoptotic stimuli, dead cells show strong fluorescence depending on caspase activation. With these tools, we monitor in real-time caspase-3-like activity in each cell under various conditions, and show for the first time that the environment of cancer cells affects their sensitivity to chemotherapeutic drugs in a modified soft agar assay. These biosensors should enable better understanding of the biological relevance of caspase-3-like proteases. Apoptosis is an essential event for animal development, and defective apoptotic processes have been implicated in an extensive variety of diseases [1] , [2] , [3] . Therefore, developing strategies to control apoptosis is a potential method for the treatment of apoptosis-associated diseases. As cytosolic caspases, such as caspase-3 and -7, have a central role in mediating the progression of apoptosis, the establishment of a rapid, convenient and reliable detection system to assess such caspases activation in various conditions is strongly desired. Recently, several sorts of noninvasive reporters to monitor caspases activation have been developed. One method is the use of fluorescence resonance energy transfer (FRET) pairs linked by peptides containing caspases cleavage sequences, such as DEVD for caspase-3 and -7. This sort of reporter is a valuable tool for studying the activity of caspases in single live cells in real-time [4] , [5] , [6] , [7] . However, the FRET-based fluorescence changes are very small. Moreover, as these reporters depend on calculated fluorescence intensity, they are largely affected by the cultural environment and cellular morphological change so that they are unlikely to be used to monitor apoptosis in a population of cells or in three-dimensional (3D) cell culture platforms. In addition, some other apoptosis reporters based on dark-to-bright fluorescence [8] or translocation of fluorescent proteins [9] have also been reported, and they require intercontrol fluorescence or depend on the spatial location of fluorescent proteins that leads to limited sensitivity and inconvenience. Another sort of reporter is derived from luciferase [10] . It requires the addition of luciferin or its derivatives, and as such it is not really a noninvasive method, in particular, it is not favourable for cell culture. The addition of chemical compounds usually terminates the cellular experiments, and thus this method is applied with difficulty in the consecutive monitoring of apoptosis. Moreover, it is difficult for luciferase-based sensors to monitor apoptosis in single live cells. All these methods require sophisticated techniques or instruments, and therefore, they are limited in practical application. To address these problems, we develop a genetically encoded switch-on fluorescence-based caspase-3-like protease activity indicator (SFCAI) generated by means of fused Npu DnaE intein. This cyclized protein contains a caspase-3 cleavage site and acquires fluorescent activity only after cleavage by activated caspase-3-like proteases. Using this tool, we measure in real-time apoptosis of each cell under various culture conditions without any addition and damaging sample. Generation of caspase-3-like protease activation indicators In order to conveniently measure the activity of caspase-3-like proteases (DEVDases), such as caspase-3 and 7 in cells, we generated a chimeric fluorescent protein whose fluorescent function was only switched on by DEVDases as caspase activity indicator (C3AI) ( Fig. 1a and Supplementary Fig. S1 ). Here we used Venus, a fast-folding variant of EYFP [11] , [12] , as the template. We first truncated the N- and C-termini of Venus and then linked them with the DEVDG polypeptide that is cleaved by DEVDases between D and G. We also generated new N′- and C′-terminal ends at Venus residues A154 and D155, and this circularly permuted short Venus could be a C3AI candidate. After cleavage by DEVDases, two fragments from the C3AI candidate have the potential to form a functional fluorescent protein based on bimolecular fluorescence complementation (BiFC) [13] ( Supplementary Fig. S1b ). To enhance the efficient complementation of the cleaved fragments of Venus, we fused a split Npu DnaE intein to the two ends of the C3AI candidate ( Fig. 1a and Supplementary Fig. S1a ). Npu DnaE intein consists of two separate polypeptides, N- and C fragments, and it can catalyze trans -ligation of its artificial exteins [14] , [15] . The ligation of N′- and C′ ends led to the cyclization of the C3AI candidate that contained additional amino acids between A154 and D155 residues. As shown in Fig. 1a , upon DEVDase cleavage, the cyclized C3AI was actually converted to a linear shortened Venus with an insertion between A154 and D155 that did not influence the fluorescent function of Venus [13] , [16] . 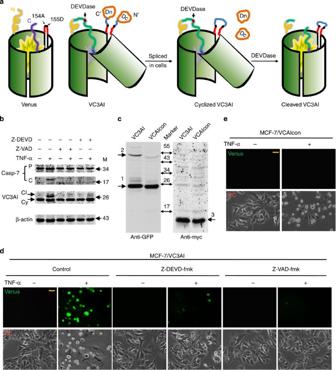Figure 1: Generation and characterization of caspase-3-like protease activity indicator. (a) Scheme for the generation of Venus-based caspase-3-like protease activity indicator (C3AI). Yellow line and purple line represent the sequences outside of the β-barrel structure (11–229 residues); green line, the cleavage sequence of caspase-3, represents the peptide sequence DEVDG; blue line means the addition insertion sequences of GSAEY and CFNEF. Dn and Dc, the N- and C fragments ofNpuDnaE intein. (b) Western analysis of levels of caspase-7, VC3AI and β-actin in MCF-7/VC3AI cells after treatments with 50 ng ml−1of TNF-α or control for 24 h in the presence or absence of 100 μM of Z-DEVD-fmk or Z-VAD-fmk (pre-treatment for 1 h). P, pro-caspase-7; C, cleaved caspase-7; Cl, cleaved VC3AI; Cy, cyclized VC3AI; M, protein marker. (c) Western analysis of the levels of VC3AI and VCAIcon in MCF-7 cells stably expressing VC3AI or VCAIcon. Both VC3AI and VCAIcon were tagged with myc epitope at the Dc domain. Band 1, cyclized VC3AI or VCAIcon (<27 kd); Band 2, possible cyclized bimolecular VC3AI or VCAIcon (<54 kd); Band 3, myc-tagged Dc fragment (13 kd). (d) The fluorescence of MCF-7/VC3AI cells after treatments as described inb. Venus, images in GFP channel; PC, phase-contrast images. (e) The fluorescence of MCF-7/VCAIcon after treatments with 50 ng ml−1of TNF-α or control for 24 h. Scale bar in all panels, 20 μm. Figure 1: Generation and characterization of caspase-3-like protease activity indicator. ( a ) Scheme for the generation of Venus-based caspase-3-like protease activity indicator (C3AI). Yellow line and purple line represent the sequences outside of the β-barrel structure (11–229 residues); green line, the cleavage sequence of caspase-3, represents the peptide sequence DEVDG; blue line means the addition insertion sequences of GSAEY and CFNEF. Dn and Dc, the N- and C fragments of Npu DnaE intein. ( b ) Western analysis of levels of caspase-7, VC3AI and β-actin in MCF-7/VC3AI cells after treatments with 50 ng ml −1 of TNF-α or control for 24 h in the presence or absence of 100 μM of Z-DEVD-fmk or Z-VAD-fmk (pre-treatment for 1 h). P, pro-caspase-7; C, cleaved caspase-7; Cl, cleaved VC3AI; Cy, cyclized VC3AI; M, protein marker. ( c ) Western analysis of the levels of VC3AI and VCAIcon in MCF-7 cells stably expressing VC3AI or VCAIcon. Both VC3AI and VCAIcon were tagged with myc epitope at the Dc domain. Band 1, cyclized VC3AI or VCAIcon (<27 kd); Band 2, possible cyclized bimolecular VC3AI or VCAIcon (<54 kd); Band 3, myc-tagged Dc fragment (13 kd). ( d ) The fluorescence of MCF-7/VC3AI cells after treatments as described in b . Venus, images in GFP channel; PC, phase-contrast images. ( e ) The fluorescence of MCF-7/VCAIcon after treatments with 50 ng ml −1 of TNF-α or control for 24 h. Scale bar in all panels, 20 μm. Full size image To obtain a robust fluorescent protein with a short sequence, we used a series of primers to truncate Venus cDNA from its two ends, and found that the deletion of the N-terminal residues 1–10 and C-terminal residues 230–238 outside of the β-barrel structure (11–229 residues) did not significantly affect fluorescence compared to the full-length construct ( Supplementary Table S1 ). Therefore, based on these deletion constructs that contained the intact β-barrel structure of Venus, we created a library of candidate constructs for C3AI ( Supplementary Table S2 and Supplementary Fig. S1a ). After being transfected into 293T cells, 11 constructs were found to have little or no fluorescent function in live cells ( Supplementary Table S2 ). Furthermore, we tested the sensitivity of these C3AI candidates to apoptosis in stable cell lines using TNF-α that induces apoptosis by an extrinsic pathway [17] , [18] . Among several cell lines tested, including HeLa, MCF-7, DU145, A549 and ACHN cells, only MCF-7 cells underwent cell death in response to TNF-α alone. MCF-7 cells were deficient in caspase-3, and thus did not display some of the typical apoptotic characteristics, such as DNA fragmentation and cellular blebbing [19] , [20] , but they still underwent morphological apoptosis upon stimuli including TNF-α treatment [21] , [22] , [23] . In addition, most of the apoptotic MCF-7 cells induced by TNF-α did not detach from the culture platform, as shown in this study, and thus MCF-7 cell line possibly was an ideal model for fluorescence-based screening using microscopy. Caspase-7, a caspase-3-like DEVDase, was cleaved and activated by TNF-α treatment, and its activation was largely repressed by a specific DEVDase inhibitor, Z-DEVD-fmk and a pan-caspase inhibitor, Z-VAD-fmk ( Fig. 1b ), suggesting that caspase-7 had an important role as an apoptotic effector in MCF-7 cells, consistent with previous reports [20] , [24] . We stably expressed all these C3AI candidates in MCF-7 cells, and found that VF5-C3AI1, VF6-C3AI1, VF7-C3AI1, VF8-C3AI1 and VF6G1-C3AI1 exhibited the highest fluorescent response to TNF-α-induced apoptosis ( Supplementary Fig. S2a ). We used VF8-C3AI1, designated hereafter as VC3AI (Venus-based C3AI), for the ongoing experiments because it contained the shortest linker that could eliminate the background fluorescence of C3AI to the most extent. As shown in Supplementary Fig. S2b , even under the high exposure of 10 s, MCF-7/VC3AI cells did not display any detectable fluorescence. This was further confirmed by the flow cytometery result that both MCF-7/wt and MCF-7/VC3AI cells almost had the same background fluorescence ( Supplementary Fig. S2c ). We generated a control, termed VCAIcon, for VC3AI by replacing DEVDG with GSGCG. Stably expressed in MCF-7 cells, VC3AI and VCAIcon proteins were almost totally cyclized by the integrated Npu DnaE intein, as indicated by the complete release of an myc-tagged N fragment of the DnaE intein (13 kd, Band 3 in Fig. 1c ), disappearance of the unspliced VC3AI fused with a myc-tagged intein (45 kd) and production of cyclized VC3AI (<27 kd, Band 1 in Fig. 1c ) that migrated a little faster than its linear counterpart (27 kd). However, we also observed an unexpected Band 2 detected by GFP antibody, and as it was not detected with a myc antibody, it could be a cyclized bimolecular VC3AI (<54 kd) that, theoretically, could also work as a biosensor like the cyclized single VC3AI. In contrast, linear VC3AI without Npu DnaE intein fusion (LVC3AI) showed detectable background fluorescence with increased protein expression ( Supplementary Fig. S3a,b ), suggesting the presence of intermolecular BiFC at high levels of LVC3AI that produced fluorescence ( Supplementary Fig. S1b ). Moreover, LVC3AI was less sensitive to TNF-α-induced apoptosis ( Supplementary Fig. S3c ) compared with VC3AI ( Fig. 1d ). It should be noted that cyclized VC3AI did not undergo intermolecular BiFC due to its structural constriction. Therefore, cyclization was indispensable for VC3AI to be a successful indicator of DEVDase activation. Cleaved VC3AI can be identified from cyclized VC3AI by western blot due to its slower mobility. In response to TNF-α, cells expressing VC3AI showed an apoptosis-associated cleavage and fluorescence, which was significantly inhibited by Z-VAD-fmk and Z-DEVD-fmk ( Fig. 1b and Supplementary Fig. S4a,b ), while MCF-7/VCAIcon cells remained non-fluorescent throughout ( Fig. 1e ). Z-DEVD-fmk is a specific irreversible inhibitor of DEVDases based on their cleavage site, tetra-peptide sequence of DEVD. It exerted a dose-dependent protective effect on TNF-α-induced fluorescence in MCF-7/VC3AI cells and almost totally blocked the fluorescence at 200 μM ( Supplementary Fig. S4a,b ). These results demonstrated that VC3AI was a specific indicator of DEVDases activity. DEVDases usually included caspase-3 and -7, while MCF-7 was deficient in caspase-3, so caspase-7 was most probably responsible for VC3AI cleavage in MCF-7 cells. This was confirmed by further results that knockdown of caspase-7 significantly suppressed TNF-α-induced fluorescence in MCF-7 cells ( Supplementary Fig. S4d–f ). VC3AI faithfully indicates TNF-α-induced apoptosis in cells TNF-α co-treatment with cycloheximide (CHX) significantly triggered cell death ( Fig. 2a ), consistent with previous reports [4] , [25] . Strong fluorescence was also observed in HeLa/VC3AI cells treated with TNF-α/CHX, and both death and fluorescence were blocked by Z-VAD-fmk ( Fig. 2a ). Western blot analysis showed that caspase-3 and 7 in HeLa/VC3AI cells treated with TNF-α/CHX were activated concomitantly with the cleavage of VC3AI and this response was attenuated by Z-VAD-fmk ( Fig. 2b ). Caspase-3/7 and VC3AI were synchronously activated during TNF-α/CHX-induced apoptosis ( Fig. 2c ), and these changes correlated with the increased number of fluorescent cells ( Fig. 2d ). Similar results were also obtained for MCF-7/VC3AI cells ( Fig. 1b and Supplementary Fig. S5 ). These results strongly suggested that the observed fluorescence of VC3AI accurately reflected the activation of DEVDases and caspases-dependent cell death. We compared the TNF-α-induced cell death between MCF-7/VC3AI and MCF-7/wt based on nuclear Hoechst staining, and no difference was observed for both MCF-7 cell lines ( Fig. 2e ), suggesting VC3AI expression did not influence cell death. 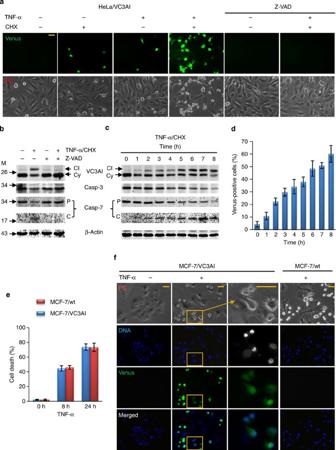Figure 2: Association of VC3AI fluorescence with apoptosis in cells. (a) The fluorescence of HeLa/VC3AI cells after treatments with 50 ng ml−1of TNF-α and/or 10 μg ml−1of CHX or control for 8 h in the presence or absence of 100 μM of Z-VAD-fmk (pre-treatment for 1 h). (b) Western analysis of levels of caspase-7, caspase-3, VC3AI and β-actin in HeLa/VC3AI cells after treatments with 50 ng ml−1of TNF-α/10 μg ml−1of CHX or control for 5 h in the presence or absence of 100 μM of Z-VAD-fmk (pre-treatment for 1 h). P, pro-caspase-7; C, cleaved caspase-7; Cl, cleaved VC3AI; Cy, cyclized VC3AI; M, protein marker. (c) Western analysis of levels of caspase-7, caspase-3, VC3AI and β-actin in HeLa/VC3AI cells after treatment with 50 ng ml−1of TNF-α/10 μg ml−1of CHX for different time as indicated. (d) The fraction of Venus-positive HeLa/VC3AI cells after treatment as described in (c). Error bar indicates ±s.d. (n=5). (e) The fraction of dead cells of MCF-7/wt and MCF-7/VC3AI cells after treatment with 50 ng ml−1of TNF-α for 8 h or 24 h. Error bar indicates ±s.d. (n=5). (f) Fluorescence images of the fixed MCF-7/wt and MCF-7/VC3AI cells after treatment with 50 ng ml−1of TNF-α for 24 h and staining with Hoechst 33258. The boxed regions are expanded in the right. PC, phase-contrast images; merged, images in GFP channel merged with those in DAPI channel. Scale bar in all panels, 20 μm. Figure 2: Association of VC3AI fluorescence with apoptosis in cells. ( a ) The fluorescence of HeLa/VC3AI cells after treatments with 50 ng ml −1 of TNF-α and/or 10 μg ml −1 of CHX or control for 8 h in the presence or absence of 100 μM of Z-VAD-fmk (pre-treatment for 1 h). ( b ) Western analysis of levels of caspase-7, caspase-3, VC3AI and β-actin in HeLa/VC3AI cells after treatments with 50 ng ml −1 of TNF-α/10 μg ml −1 of CHX or control for 5 h in the presence or absence of 100 μM of Z-VAD-fmk (pre-treatment for 1 h). P, pro-caspase-7; C, cleaved caspase-7; Cl, cleaved VC3AI; Cy, cyclized VC3AI; M, protein marker. ( c ) Western analysis of levels of caspase-7, caspase-3, VC3AI and β-actin in HeLa/VC3AI cells after treatment with 50 ng ml −1 of TNF-α/10 μg ml −1 of CHX for different time as indicated. ( d ) The fraction of Venus-positive HeLa/VC3AI cells after treatment as described in ( c ). Error bar indicates ±s.d. ( n =5). ( e ) The fraction of dead cells of MCF-7/wt and MCF-7/VC3AI cells after treatment with 50 ng ml −1 of TNF-α for 8 h or 24 h. Error bar indicates ±s.d. ( n =5). ( f ) Fluorescence images of the fixed MCF-7/wt and MCF-7/VC3AI cells after treatment with 50 ng ml −1 of TNF-α for 24 h and staining with Hoechst 33258. The boxed regions are expanded in the right. PC, phase-contrast images; merged, images in GFP channel merged with those in DAPI channel. Scale bar in all panels, 20 μm. Full size image To further confirm the correlation between the fluorescence of VC3AI and TNF-α-induced apoptosis, we merged fluorescence from VC3AI and DNA staining, and found that nuclear chromatin condensation occurred only in Venus-positive cells ( Figs 2f and 3a ). This indicated that VC3AI fluorescence faithfully reflected TNF-α-induced death in MCF-7/VC3AI cells. In addition, we found that a fraction of Venus-positive cells had similar cellular morphology to the control, although these Venus-positive cells had condensed nuclear DNA and altered nuclear shape ( Fig. 2f ), especially in MCF-7/VC3AI cells treated for 8 h with TNF-α ( Fig. 3a ). In contrast, the morphology of HeLa cells treated with TNF-α/CHX changed significantly with most of the apoptotic cells having blebs or apoptotic bodies ( Fig. 2a and Supplementary Fig. S6a ). Moreover, some of the HeLa/VC3AI cells floated in the buffer, and most of these were fluorescence-positive ( Supplementary Fig. S6a ). However, we still observed some Venus-positive HeLa/VC3AI cells with normal morphology after 8-h treatment with TNF-α/CHX ( Fig. 2a and Supplementary Fig. S6b ). These may represent cells in very early stages of apoptosis. 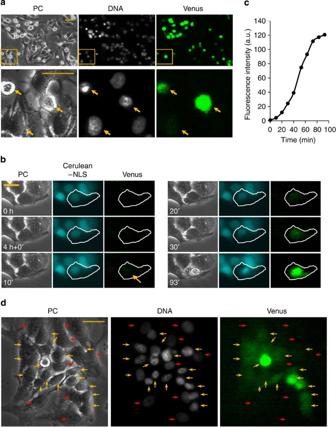Figure 3: Real-time fluorescence of VC3AI in apoptotic cells. (a) Fluorescence of the fixed MCF-7/VC3AI cells after treatment with 50 ng ml−1of TNF-α for 8 h. The boxed regions are expanded in the right. Arrow shows fluorescent cells. (b) MCF-7 cells stably expressing VC3AI and Cerulean-NLS were seeded in the six-well plate. After they were treated with 50 ng ml−1of TNF-α for 4 h, cells in the fixed region were imaged at intervals at room temperature. Arrow shows the emergence of the fluorescence from VC3AI. (c) Fluorescence intensity of MCF-7/VC3AI cells versus time. Data are calculated fromb. (d) Fluorescence of the fixed MCF-7/VC3AI cells after treatments with 50 ng ml−1of TNF-α for 24 h in the presence of 50 μM of Z-DEVD-fmk (pre-treatment for 1 h). Yellow and red arrows show fluorescent and non-fluorescent cells, respectively. Scale bar in all panels, 20 μm. Figure 3: Real-time fluorescence of VC3AI in apoptotic cells. ( a ) Fluorescence of the fixed MCF-7/VC3AI cells after treatment with 50 ng ml −1 of TNF-α for 8 h. The boxed regions are expanded in the right. Arrow shows fluorescent cells. ( b ) MCF-7 cells stably expressing VC3AI and Cerulean-NLS were seeded in the six-well plate. After they were treated with 50 ng ml −1 of TNF-α for 4 h, cells in the fixed region were imaged at intervals at room temperature. Arrow shows the emergence of the fluorescence from VC3AI. ( c ) Fluorescence intensity of MCF-7/VC3AI cells versus time. Data are calculated from b . ( d ) Fluorescence of the fixed MCF-7/VC3AI cells after treatments with 50 ng ml −1 of TNF-α for 24 h in the presence of 50 μM of Z-DEVD-fmk (pre-treatment for 1 h). Yellow and red arrows show fluorescent and non-fluorescent cells, respectively. Scale bar in all panels, 20 μm. Full size image Real-time measurement of apoptosis in single live cells To confirm whether VC3AI fluorescence is a very early apoptotic indicator and useful in detecting real-time caspase-dependent cell death, we monitored apoptotic events at the same time, such as nuclear morphological changes using a nucleus-localizing form of Cerulean (Cerulean-NLS), cellular morphology under bright field and caspases activation by fluorescence from VC3AI. MCF-7 cells expressing VC3AI and Cerulean-NLS were treated with TNF-α for 4 hours, and cells were imaged at different time points. As shown in Fig. 3b , TNF-α-induced VC3AI fluorescence in MCF-7 cells preceded the significant changes in the nuclear and cellular morphology by about 10 min, and a similar delay was also observed in the previous report [4] . This was consistent with the results in Figs 2f and 3a and Supplementary Fig. S6b . Furthermore, the kinetics of fluorescence showed that the full activation of VC3AI required ~70 min ( Fig. 3c ), comparable to the previously reported 90 min for FRET-based apoptosis reporter in MCF-7 cells [6] . Venus, the precursor of VC3AI, is able to immediately mature to a fully functional fluorescent protein [12] . Cleaved VC3AI could potentially mature faster than Venus, as the fluorescent chromophore in the folded N-terminal fragment may already be formed [26] and the N- and C-fragments of cyclized VC3AI may already exist in a correctly folded state based on results using BiFC technology [16] . Therefore, VC3AI could act as a real-time monitoring tool of DEVDases activity. As an effective substrate of DEVDase, the cleaved VC3AI could accumulate over time and thus indicate DEVDases with low activity. We observed that, in the presence of a low concentration of Z-DEVD-fmk (50 μM), not only the number of fluorescent MCF-7/VC3AI cells but also the fluorescence intensity significantly decreased upon TNF-α treatment ( Supplementary Fig. S4a,b,c ). Almost all the fluorescent cells contained condensed chromatin but most of them had relatively normal cellular and nuclear morphology ( Fig. 3d ). The similar phenomenon was also observed in HeLa/VC3AI cells ( Supplementary Fig. S6c ). This not only confirmed that VC3AI fluorescence preceded the significant morphological changes during TNF-α-induced apoptosis, but also suggested that VC3AI could detect a low level of activated DEVDases. VC3AI reveals distinct responses to chemotherapeutic drugs We tested the response of MCF-7/VC3AI cells to two commonly used anticancer drugs, 5-fluorouracil (5-FU) and cisplatin. 5-FU showed a marginal killing effect on MCF-7/VC3AI cells after 24 h treatment. Even at a concentration of 1 mg ml −1 , it only induced apoptosis in ~27% of cells based on the number of fluorescence-positive cells and this was similar to the number of dead cells measured using Hoechst 33258 staining ( Fig. 4a ). Interestingly, we observed numerous fluorescence-positive MCF-7/VC3AI cells that had normal cellular and nuclear morphology but their chromatins were virtually condensed ( Fig. 4b ), similar to TNF-α-treated MCF-7/VC3AI cells ( Figs 2f and 3a ). We also observed similar responses in HeLa/VC3AI cells ( Fig. 5a and Supplementary Fig. S7 ). Therefore, given the dose of the drug and the time of exposure, these cells are most probably in the early stages of apoptosis. Furthermore, we observed that although all fluorescence-positive HeLa/VC3AI cells treated with 5-FU had condensed chromatins, many of the cells had more than one nucleus ( Fig. 5a and Supplementary Fig. S7 ), in contrast to MCF-7/VC3AI cells ( Fig. 4b ), suggesting that 5-FU altered cell cycle progression before inducing apoptosis. 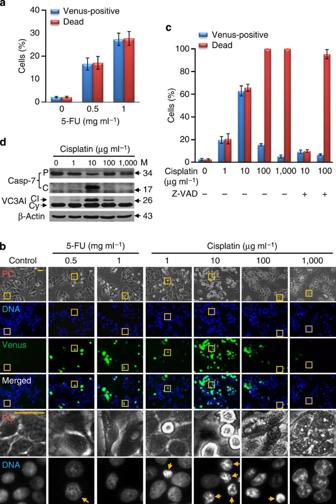Figure 4: Response of VC3AI in MCF-7 cells to chemotherapeutical drugs. (a) The fractions of dead and Venus-positive MCF-7/VC3AI cells after treatment with 5-FU for 24 h. Error bar indicates ±s.d. (n=5). (b) Fluorescence of MCF-7/VC3AI cells after treatment with 5-FU or cisplatin for 24 h. The boxed regions are expanded in the two rows at the bottom. PC, phase-contrast images; merged, images in GFP channel merged with those in DAPI channel. Arrows show apoptotic cells. Scale bar, 20 μm. (c) The fractions of dead and Venus-positive MCF-7/VC3AI cells after treatments with cisplatin in the presence or absence of 100 μM of Z-VAD-fmk for 24 h. Error bar indicates ±s.d. (n=5). (d) Western analysis of levels of caspase-7, VC3AI and β-actin in MCF-7/VC3AI cells after treatment with cisplatin for 5 h. P, pro-caspase-7; C, cleaved caspase-7; Cl, cleaved VC3AI; Cy, cyclized VC3AI; M, protein marker. Figure 4: Response of VC3AI in MCF-7 cells to chemotherapeutical drugs. ( a ) The fractions of dead and Venus-positive MCF-7/VC3AI cells after treatment with 5-FU for 24 h. Error bar indicates ±s.d. ( n =5). ( b ) Fluorescence of MCF-7/VC3AI cells after treatment with 5-FU or cisplatin for 24 h. The boxed regions are expanded in the two rows at the bottom. PC, phase-contrast images; merged, images in GFP channel merged with those in DAPI channel. Arrows show apoptotic cells. Scale bar, 20 μm. ( c ) The fractions of dead and Venus-positive MCF-7/VC3AI cells after treatments with cisplatin in the presence or absence of 100 μM of Z-VAD-fmk for 24 h. Error bar indicates ±s.d. ( n =5). ( d ) Western analysis of levels of caspase-7, VC3AI and β-actin in MCF-7/VC3AI cells after treatment with cisplatin for 5 h. P, pro-caspase-7; C, cleaved caspase-7; Cl, cleaved VC3AI; Cy, cyclized VC3AI; M, protein marker. 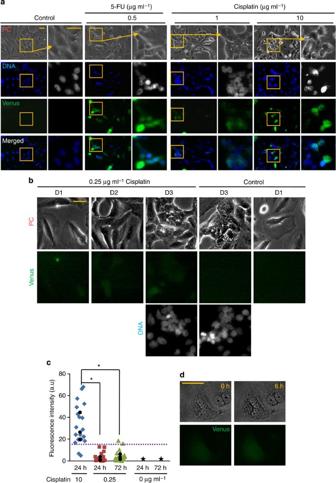Figure 5: Response of VC3AI in HeLa/VC3AI Cells to anticancer drugs. (a) Fluorescence of HeLa/VC3AI cells after treatment with 5-FU or cisplatin for 24 h. The boxed regions are expanded in the right. PC, phase-contrast image; merged, the images in GFP channel are merged with those in DAPI channel (DNA). (b) Fluorescence of HeLa/VC3AI cells after treatment with 0.25 μg ml−1of cisplatin for different time. Cells with ‘condensed chromatin’ should be undergoing division. (c) Scatter plot showing the fluorescence intensity of MCF-7/VC3AI cells after treatment with cisplatin as indicated. Black symbols represent first quartile, median and third quartile. *P<0.01 (- test,n=20).★, no detectable fluorescence over background. (d) Fluorescence of HeLa/VC3AI cells in the fixed region treated with 0.25 μg ml−1of cisplatin for 2 days at intervals as indicated. Scale bar in all panels, 20 μm. Full size image Figure 5: Response of VC3AI in HeLa/VC3AI Cells to anticancer drugs. ( a ) Fluorescence of HeLa/VC3AI cells after treatment with 5-FU or cisplatin for 24 h. The boxed regions are expanded in the right. PC, phase-contrast image; merged, the images in GFP channel are merged with those in DAPI channel (DNA). ( b ) Fluorescence of HeLa/VC3AI cells after treatment with 0.25 μg ml −1 of cisplatin for different time. Cells with ‘condensed chromatin’ should be undergoing division. ( c ) Scatter plot showing the fluorescence intensity of MCF-7/VC3AI cells after treatment with cisplatin as indicated. Black symbols represent first quartile, median and third quartile. * P <0.01 (- test, n =20). ★ , no detectable fluorescence over background. ( d ) Fluorescence of HeLa/VC3AI cells in the fixed region treated with 0.25 μg ml −1 of cisplatin for 2 days at intervals as indicated. Scale bar in all panels, 20 μm. Full size image Cisplatin exerted a potent killing effect on MCF-7 cells and it induced apoptosis, respectively, in 20 and 65% of cells at the concentrations of 1 μg ml −1 and 10 μg ml −1 after 24-h treatment ( Fig. 4c ). The fluorescence-positive cells were almost identical to the dead ones ( Fig. 4b ). Interestingly, higher concentrations of cisplatin (100 and 1,000 μg ml −1 ) had lower apoptosis-inducing ability based on fluorescence induction in cells, and a concentration of 1,000 μg ml −1 of cisplatin almost completely failed to activate VC3AI, although it still killed all MCF-7 cells ( Fig. 4b ). At these high doses, cellular morphology changed significantly, the cytoplasmic membrane seemed to breakdown, nuclear shape was not altered greatly, but nuclear chromatin intensity decreased ( Fig. 4b ). Furthermore, the cell death induced by a high concentration of cisplatin (100 μg ml −1 ) was not rescued by Z-VAD, while death by low concentration (10 μg ml −1 ) was blocked by Z-VAD ( Fig. 4c ), suggesting a necrotic cell death in MCF-7/VC3AI treated with a high concentration of cisplatin. These results suggested that cisplatin triggered apoptosis at low concentrations but necrosis at high concentrations in MCF-7 cells. In the meantime, we examined the effect of cisplatin treatment of cells on the cleavage of VC3AI and caspases. Activation of caspase-7 and the cleavage of VC3AI were synchronous upon cisplatin treatment, but cisplatin at a high concentration did not activate caspase-7 and VC3AI ( Fig. 4d ). Cisplatin was also toxic to HeLa cells at high concentrations (100 and 1,000 μg ml −1 ), and most of the dead cells were fluorescence-negative ( Supplementary Fig. S7 ), whereas HeLa/VC3AI cells treated with cisplatin at 1 or 10 μg ml −1 had robust fluorescence and condensed chromatins ( Fig. 5a ). Like 5-FU, cisplatin also produced multinucleated HeLa cells, which was associated with the activated VC3AI fluorescence and chromatin condensation ( Fig. 5a and Supplementary Fig. S7 ). It appears that HeLa cells became multinucleated when their cell cycle was disturbed and then underwent apoptosis. Taken together, the cell death and resulting biological events of cancer cells depended very much on the stimuli and cell types. It should be noted that all dead cells induced by stimuli including TNF-α/CHX contained a fraction of fluorescence-negative cells, with the exception of MCF-7/VC3AI cells treated with TNF-α alone where dead cells were identical to the fluorescent ones ( Figs 2 , 3 , 4 , 5 , Supplementary Figs S6 and S7a ). The number of fluorescence-negative dead cells increased with the concentrations of chemical stimuli ( Figs 4 and 5 , Supplementary Fig. S7a ). This suggested the presence of non-apoptotic cell death induced by clinical drugs, although these compounds were previously reported to specifically elicit apoptosis. VC3AI fluorescence was a reliable indicator of apoptosis in the dead cell population and thus revealed discrepancies between cell death and apoptosis. VC3AI can detect DEVDases activity in non-dying cells Our forenamed results ( Fig. 3d and Supplementary Fig. S4a,b ) showed that VC3AI can detect DEVDases with low activity that were implicated in the non-apoptotic cells and are required for normal cell survival in some conditions [27] , [28] , [29] , [30] . Therefore, we investigated whether DEVDase can be slightly activated in cancer cells without death induction. We treated HeLa/VC3AI cells with different concentrations of cisplatin (0.05, 0.1, 0.25, 0.5 and 1 μg ml −1 ) for days. In fact, low concentrations of cisplatin (<0.5 μg ml −1 ) showed no effect on HeLa/VC3AI cells at least during 3 days; however, some fluorescent cells were clearly observed when HeLa/VC3AI cells were treated with 0.25 μg ml −1 of cisplatin and they had relatively normal nuclear chromatin, compared with the control HeLa/VC3AI cells ( Fig. 5b ). The fluorescence intensity induced by 0.25 μg ml −1 of cisplatin was much weaker than that by 10 μg ml −1 of cisplatin that induced apoptosis ( Fig. 5c ). To further explore whether these fluorescent cells were undergoing apoptosis in the very early stages, we followed the fluorescent cells in one area for 6 h, and no obviously morphological change was observed ( Fig. 5d ), suggesting no apoptosis. Although some of the HeLa/VC3AI cells treated with TNF-α/CHX plus 50 μM of z-DEVD-fmk also showed fluorescence without morphological change during 24 h ( Supplementary Figs S6c and S7b ), they finally underwent substantial morphological apoptosis after 48 h treatments ( Supplementary Fig. S7b ). Driven by the upstream apoptotic signals triggered by TNF-α/CHX, the residual active DEVDases, though partially inhibited by z-DEVD-fmk, continuously elicited downstream apoptotic events accompanied by increased fluorescence intensity ( Supplementary Fig. S7b,c ), which eventually led to morphological apoptosis. In contrast, the fluorescence intensity of HeLa/VC3AI cells under mild chemical stress did not increase with time ( Fig. 5c ). Therefore, DEVDases in HeLa/VC3AI cells possibly were transiently activated under the condition of mild chemical stress. VC3AI indicates apoptosis in soft agar assay Anchorage-independent growth in soft agar is one of the hallmark characteristics of cellular transformation. Moreover, as one of the 3D formats for cell growth, soft agar cell culture is considered superior to monolayer cell culture in drug testing [31] . However, it can be difficult to assay for cell death in soft agar, and this limited the application of this culture format. Here we tested the use of VC3AI to detect apoptosis in cells in the soft agar. HeLa/VC3AI and MCF-7/VC3AI cells were seeded into the top soft agar, and then colony formation was monitored by fluorescence microscopy. As only a portion of plated cells have the ability to form robust colonies after plating in agar, we expected to observe some cell death after plating. As shown in Supplementary Fig. S8a , some HeLa/VC3AI cells (a′) were apoptotic after seeding at Day 0 as indicated by fluorescence, while some cells (b′) grew to form a colony that started to show fluorescence at Day 6 and then stopped growing. One colony of MCF-7/VC3AI (d′) showed strong fluorescence and then stopped growing at Day 7, while another colony (c′) without fluorescence continued to grow ( Supplementary Fig. S8b ). These results showed that VC3AI was useful for the detection of apoptosis in a soft agar assay. To test the sensitivity of cells in the colony (diameter >50 μm) to anticancer drugs, medium containing cisplatin was added onto the top of the agarose layer. After treatment with 10 μg ml −1 of cisplatin for 24 h, 26.7% of colonies were fluorescent, compared with 8.6% in the control ( Fig. 6a ). Moreover, fluorescence was observed only in part of the colony after 24 h but fluorescence expanded to the whole colony over time ( Fig. 6b ). 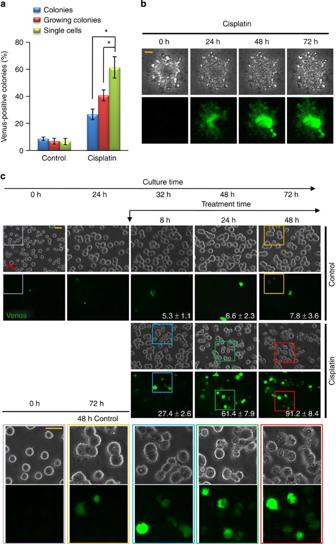Figure 6: Detection of apoptosis in soft agar by VC3AI. (a) The fractions of fluorescence-positive colonies of MCF-7/VC3AI cells after treatment with 10 μg ml−1of cisplatin for 24 h. Colonies: diameters >50 μm after cells grew in soft agar for 3 weeks; growing colonies: diameters are around 20 μm after cells grew in the modified soft agar for one week; single cells: cells were seeded in the modified soft agar for 24 h. Error bar indicates ±s.d. (n=5). *P<0.05 (t-test). (b) Fluorescence of one MCF-7/VC3AI colony in the soft agar after treatment with 10 μg ml−1of cisplatin for different time. (c) Fluorescence of MCF-7/VC3AI cells seeded in the same layer in the modified soft agar assay. After being cultured for 24 h, they were treated with 10 μg ml−1of cisplatin for different time periods. The regions in the coloured boxes are expanded at the bottom, respectively. The numbers in fluorescent images are the percentages of fluorescence-positive cells (means±s.d.,n=5). Scale bar in all panels, 20 μm. Figure 6: Detection of apoptosis in soft agar by VC3AI. ( a ) The fractions of fluorescence-positive colonies of MCF-7/VC3AI cells after treatment with 10 μg ml −1 of cisplatin for 24 h. Colonies: diameters >50 μm after cells grew in soft agar for 3 weeks; growing colonies: diameters are around 20 μm after cells grew in the modified soft agar for one week; single cells: cells were seeded in the modified soft agar for 24 h. Error bar indicates ±s.d. ( n =5). * P <0.05 ( t -test). ( b ) Fluorescence of one MCF-7/VC3AI colony in the soft agar after treatment with 10 μg ml −1 of cisplatin for different time. ( c ) Fluorescence of MCF-7/VC3AI cells seeded in the same layer in the modified soft agar assay. After being cultured for 24 h, they were treated with 10 μg ml −1 of cisplatin for different time periods. The regions in the coloured boxes are expanded at the bottom, respectively. The numbers in fluorescent images are the percentages of fluorescence-positive cells (means±s.d., n =5). Scale bar in all panels, 20 μm. Full size image To determine the sensitivity of single MCF-7 cells to cisplatin in the soft agar culture platform, we seeded MCF-7/VC3AI cells in the same layer between top and bottom agarose, and both agarose layers were 0.3%, as previously described [32] . This modified soft agar assay allowed us to easily focus on a population of cells, like the two-dimensional (2D) cell culture. After cells were cultured for 24 h, 10 μg ml −1 of cisplatin was added and it induced readily detectable fluorescence in cells and the fluorescence-positive cell number increased with treatment time with 27.4, 61.4 and 91.2% of cells being fluorescence-positive after treatment for 8, 24 and 48 h, while only 5.3, 6.6 and 7.8% of cells showed fluorescence in the controls ( Fig. 6c ). Therefore, single MCF-7/VC3AI cells in soft agar assay were more sensitive to cisplatin than cells in colonies ( Fig. 6a ), and this sensitivity was similar to that of cells in the 2D culture platform ( Figs 4c and 6a ). In addition, we also tested the sensitivity of cells in small growing colonies to cisplatin in the modified soft agar platform. MCF-7/VC3AI cells were seeded in the same layer between top and bottom agarose, and cultured for 1 week. When the cells had formed small colonies (diameters ~20 μm), we treated the cells with 10 μg ml −1 of cisplatin. After treatment for 24 h, 40.7% of the colonies were fluorescence-positive ( Fig. 6a ). Like the larger colonies (diameters >50 μm) treated with cisplatin, the growing colonies also displayed fluorescence expanding from some cells to the whole colony with time ( Supplementary Fig. S8c ). Based on the above results, the environment of MCF-7 cells affected their sensitivity to anticancer drugs. As the environment of cancer cells in vivo is variable and differs from in vitro conditions, this modified soft agar assay provides a technique to measure in vitro the sensitivity of transformed cells under various conditions to anticancer drugs. VC3AI was a very useful tool to monitor cell death in this cell culture platform. Design and testing of C3AIs based on fluorescent proteins To potentially broaden the usefulness of the technology described here, we also generated Cerulean [33] (cyan fluorescence), sfGFP [34] (a superfolder green fluorescence) and mCherry [35] (red fluorescence)-based C3AI. As Cerulean and sfGFP share similar sequence and structure to Venus, the method of generation of Cerulean-based C3AI (CC3AI) and sfGFP-based C3AI (GC3AI) indicators was the same as that of VC3AI. We generated F6-CC3AI, F8-CC3AI, F6-GC3AI and F8-GC3AI as candidates (see Supplementary Table S3 ). To generate mCherry-based RC3AI, we used DEVDG to link its shortened ends, and generated new termini at 154D–155G based on its structure and application in BiFC [36] , and fused these ends with Npu DnaE intein. We generated four candidates for RC3AI with different truncations at the N terminus: RC3AI.1, RC3AI.2, RC3AI.3 and RC3AI.4, ( Supplementary Table S3 ). We did not know why F8-CC3AI and F8-GC3AI were not well expressed in MCF-7 cells (data not shown). Therefore, F6-CC3AI and F6-GC3AI were termed CC3AI and GC3AI, and both of them showed significant fluorescence upon TNF-α-induced apoptosis ( Fig. 7a ). Among the four RC3AI candidates, RC3AI.1 and RC3AI.2 had detectable background fluorescence ( Supplementary Fig. S9 ), but RC3AI.3 and RC3AI.4 were non-fluorescent. After MCF-7/RC3AI.3 and MCF-7/RC3AI.4 cells were treated with TNF-α, red fluorescence was observed in dead cells ( Fig. 7c ). Actually, we tested the application of many fluorescent proteins, such as ECFP, EGFP, EYFP, copGFP and a far-red protein, mKate2 (ref. 37 ), in C3AI, but none of them worked (data not shown). 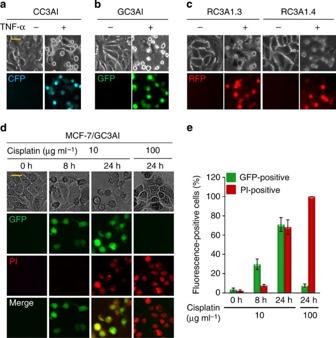Figure 7: C3AIs based on alternative fluorescent proteins. MCF-7 cells stably expressing CC3AI (a), GC3AI (b) or RC3AI (c) were treated with 50 ng ml−1of TNF-α for 24 h, and then imaged. RC3AI.3 and RC3AI.4 contain different linkers and details are given inSupplementary Table S3. (d) MCF-7/GC3AI cells were treated with cisplatin for different time periods as indicated, and then stained with PI before imaging. (e) The fraction of MCF-7/GC3AI cells with GFP or PI fluorescence after treatments as described ind. Error bar indicates ±s.d. (n=5). Scale bar in all panels, 20 μm. Figure 7: C3AIs based on alternative fluorescent proteins. MCF-7 cells stably expressing CC3AI ( a ), GC3AI ( b ) or RC3AI ( c ) were treated with 50 ng ml −1 of TNF-α for 24 h, and then imaged. RC3AI.3 and RC3AI.4 contain different linkers and details are given in Supplementary Table S3 . ( d ) MCF-7/GC3AI cells were treated with cisplatin for different time periods as indicated, and then stained with PI before imaging. ( e ) The fraction of MCF-7/GC3AI cells with GFP or PI fluorescence after treatments as described in d . Error bar indicates ±s.d. ( n =5). Scale bar in all panels, 20 μm. Full size image In BiFC technology, the N-terminal and C-terminal fragments of Venus, Cerulean and mKate efficiently complement each other at 37 °C (refs 13 , 16 , 38 ), while those of mCherry, ECFP, EGFP and EYFP did not [36] . However, when used as part of C3AI, Venus, Cerulean and mCherry worked well at the normal cell culture condition. Therefore, BiFC and cleaved C3AI possibly followed different maturing mechanisms. Indeed, cleaved C3AI was a single protein with correctly folded N- and C fragments, while BiFC actually involved two proteins. These C3AIs with different fluorescence certainly increase their compatibility with other fluorescent proteins or dyes. For example, propidium iodide (PI) is usually used to stain dead cells with permeable membrane, and its fluorescence overlaps with VC3AI but works well together with GC3AI. Our forenamed results in Fig. 4 showed that cisplatin induced apoptosis at low concentrations but necrosis at high concentrations. Here, we further confirmed this speculation in MCF-7/GC3AI cells using PI staining. After being treated with 100 μg ml −1 of cisplatin for 24 h, almost all MCF-7/GC3AI cells were GFP-negative but they were PI-positive ( Fig. 7d ), suggesting necrotic cell death. In contrast, cells treated with 10 μg ml −1 of cisplatin showed robust GFP fluorescence, and most of the fluorescent cells were PI-negative in 8-h treatment but positive after 24-h treatment ( Fig. 7d ). Taken together, GC3AI in combination with PI staining can easily distinguish cells in different states: live cells (GFP-negative and PI-negative); necrotic cells (GFP-negative; PI-positive); apoptotic cells in early stages (GFP-positive; PI-negative); apoptotic cells in late stages (GFP-positive; PI-positive). VC3AI allows real-time monitoring of apoptosis in each cell in a population of cells without addition, sample damage and sophisticated techniques or instruments. VC3AI is sensitive, because its active form with fluorescence is significantly distinct from the non-fluorescent precursor, which renders VC3AI as a very convenient and reliable indicator of apoptosis based on the emerging of fluorescence. Therefore, VC3AI is useful for cellular apoptosis detection in various conditions, such as 2D and 3D cell culture platforms. VC3AI only responds to activated caspase-3-like proteases, so it can easily distinguish apoptosis from other types of cell death, which allows veridically evaluating the apoptosis-inducing ability of treatments, and this may be very important for the testing of apoptosis-related drugs. In addition, we can expand the application of 3D cell culture platforms with VC3AI. In this study, we use a modified soft agar assay, where single cells are seeded in the same layer, to visualize apoptosis of cells following treatments like in the monolayer cell culture, and certainly reveal that the sensitivity of MCF-7 cells to cisplatin is largely affected by the cellular environment. Another potential application of VC3AI is its use in a high-throughput screening platform for antitumor drugs. Read-out of fluorescence would be a simple indicator of the apoptosis-inducing ability of candidate compounds. The fluorescent cleaved VC3AI with a half-life time of ~40 h was relatively stable ( Supplementary Fig. S10 ), and this should be adequate for most screening methods. Moreover, in view of its stability, the cleaved VC3AI may indicate a low level of active DEVDases by accumulating with time or uncover the presence of DEVDases that were once activated. This may be helpful to the studies on the non-apoptotic functions of DEVDases that had been demonstrated to occur under some conditions [27] , [28] , [29] . In addition, we also constructed apoptosis sensors based on different fluorescent proteins as complements to VC3AI to expand the application of C3AI. These C3AIs can be selectively used in experiments in combination with other fluorescent reporters. SFCAI may represent another biotechnological application of fluorescent proteins, in contrast to FRET and BiFC. SFCAI technology should be useful to measure the activity of other proteases both in vitro and in vivo . However, as the linker in the SFCAI was constrained to a specified length that inactivated the function of fluorescent protein, functioning SFCAI-based indicator depends on the specific properties of the proteases, such as the length of cleavage sequences and the structure of active sites. Gene construction All cDNAs for fluorescent protein variants were generated by PCR, and the humanized cDNA of Npu DnaE intein was commercially synthesized (Genewiz, China). All cDNAs were cloned into lentiviral expression vectors, pCDH-puro-CMV or pCDH-Neo-CMV using the eFusion Recombinant Cloning Kit (Biophay, China). The pLKO.1 lentiviral RNAi expression system was used to construct lentiviral shRNA for caspase-7. The sequences of shRNA used in this study included the following: shScramble: 5′-CCGGCCTAAGGTTAAGTCGCCCTCGCTCGAGCGAGGGCGACTTAACCTTAGGTTTTT-3′ shCaspase-7#1: 5′-CCGGGTATGTCTGTTACCTTGTTAACTCGAGTTAACAAGGTAACAGACATACTTTTT-3′ shCaspase-7#2: 5′-CCGGTACTTCAGTCAATAGCCATATCTCGAGATATGGCTATTGACTGAAGTATTTTT-3′ Cell culture Cells were maintained in DMEM (high glucose) supplemented with 10% foetal bovine serum (Hyclone, USA) and 50 IU penicillin/streptomycin (Invitrogen, USA) in a humidified atmosphere with 5% CO 2 at 37 °C. 2 × 10 5 cells per well were seeded in six-well plates for all anchorage-dependent experiments except those lasting for 3 days of treatments where 0.5 × 10 5 cells per well were seeded in six-well plates ( Fig. 5b ). Anchorage-independent cell culture For soft agar assays, 10 4 cells suspended in top agarose solution were poured over a layer of bottom agarose previously solidified in six-well plates. Cells were cultured in a humidified atmosphere with 5% CO2 at 37 °C. For the modified soft agar assay [32] , 10 5 cells in 20 μl of medium were dropped on the solidified bottom agarose in six-well plates, and then the top agarose was carefully added from one side to cover the spread cells. After agarose was solidified, cells were imaged with a Nikon Eclipse TE2000-U fluorescence microscope (Nikon, Japan) as Day 0. The top and bottom layers of agarose were 0.3% for all the experiments. The volume of top and bottom agarose layers was 1 ml. Treatments involved adding 2 ml of medium containing a double concentration of compound onto the agarose. Imaging of cultured cells For live-cell imaging, cells were grown in six-well plates, and after the desired treatments, the fluorescence and phase-contrast imaging was captured with a Nikon Eclipse TE2000-U fluorescence microscope. For fixed-cell imaging, after the desired treatments, cells grown in six-well plate were fixed with 4% paraformaldehyde in PBS for 30 min, and then carefully washed twice with PBS buffer. The fixed cells were incubated with 2 μg ml −1 of Hoechst 33258 for 5 min for nuclear DNA staining. After washing twice with PBS, the cells were imaged. The filter sets for imaging were: Venus/GFP: Ex480/30, DM505, BA535/40; RFP: Ex535/50, DM575, BA590; CFP: Ex440/21, DM455, BA480/30. The fluorescence intensity of images was analyzed with ImageJ software. Cell death assay After desired treatments, cells grown in plates were fixed, stained with Hoechst 33258 (Sigma, USA) and imaged as described above. Cells containing condensed chromatins were counted as dead. For PI staining, after desired treatments, live cells were stained with 10 μg ml −1 of PI for 10 min, and then the staining medium was carefully removed and replaced with fresh medium. Cells were imaged in RFP channel as described above. Western blot After desired treatments as specified as indicated, cells were washed twice with PBS and lysed in buffer (20 mM Tris–HCl, pH 7.5, 150 mM NaCl, 1 mM EDTA, 1% Triton X-100, 2.5 mM sodium pyrophosphate, 1 mM β-glycerophosphate, 1 mM sodium vanadate, 1 mg ml −1 leupeptin, 1 mM phenylmethyl-sulfonylfluoride). Equal amounts of protein (30 μg) were loaded onto 15% SDS–PAGE gels. Western detection was carried out using a Li-Cor Odyssey image reader (Li-Cor, USA). Anti-Caspase-3 (catalogue number: 9665), anti-Caspase-7 (catalogue number: 9494), anti-myc tag (catalogue number: 2276), anti-GFP (catalogue number: 2955) and anti-β-Actin (catalogue number: 8457) antibodies were obtained from Cell Signaling Technology (USA). All these primary antibodies were used with a dilution of 1:1,000. The goat anti-mouse immunoglobulin G (IgG) and goat anti-rabbit IgG secondary antibodies were obtained from Li-Cor (USA). The final concentration of the secondary antibodies used was 0.1 μg ml −1 . Lentivirus production Viral packaging was done according to a previously described protocol [39] . Briefly, expression plasmids pCDH-CMV-cDNA, pCMV-dR8.91 and pCMV-VSV-G were co-transfected into 293T cells using the calcium phosphate coprecipitation at 20:10:10 μg (for a 10-cm dish). The transfection medium containing calcium phosphate and plasmid mixture was replaced with fresh complete medium after incubation for 5 h. Media containing virus was collected 48 h after transfection and then concentrated using Virus Concentrator Kit (Biophay, China). The virus was resuspended in the appropriate amount of complete growth medium and stored at −80 °C. Cancer cells were infected with the viruses at the titre of 100% infection in the presence of polybrene (10 μg ml −1 ) for 48 h, and then the cells were selected with puromycin or neomycin. Statistics Data are given as means±s.d. For statistical comparison, one-way analysis of variance and Tukey’s test were used. Asterisks in the figures indicated statistical significances ( P <0.05). Assessment of cleaved VC3AI stability MCF-7/VC3AI cells were treated with 50 ng ml −1 of TNF-α for 8 h, and then TNF-α was removed and cells were incubated with 100 μM of z-VAD-fmk and 25 μg ml −1 of cycloheximide to block caspases activation and protein synthesis. The fluorescence was imaged at different times. The half-life time of cleaved VC3AI can be assessed from the plot of ‘fluorescence intensity (percentage) versus time’. How to cite this article: Zhang, J. et al . Visualization of caspase-3-like activity in cells using a genetically encoded fluorescent biosensor activated by protein cleavage. Nat. Commun. 4:2157 doi: 10.1038/ncomms3157 (2013).